Smad6 inhibits non-canonical TGF-β1 signalling by recruiting the deubiquitinase A20 to TRAF6 Transforming growth factor (TGF)-β, a pivotal cytokine involved in a variety of cellular functions, transmits signals through Smad-dependent canonical and Smad-independent noncanonical pathways. In contrast to the canonical TGF-β pathway, it is unknown how noncanonical TGF-β pathways are negatively regulated. Here we demonstrate that the inhibitory Smad Smad6, but not Smad7, negatively regulates TGF-β1-induced activation of the TRAF6-TAK1-p38 MAPK/JNK pathway, a noncanonical TGF-β pathway. TGF-β1-induced Smad6 abolishes K63-linked polyubiquitination of TRAF6 by recruiting the A20 deubiquitinating enzyme in AML-12 mouse liver cells and primary hepatocytes. In addition, the knockdown of Smad6 or A20 in an animal model or cell culture system maintains TAK1 and p38 MAPK/JNK phosphorylation and increases apoptosis, emphasizing the crucial role of the Smad6-A20 axis in negative regulation of the TGF-β1-TRAF6-TAK1-p38 MAPK/JNK pathway. Therefore, our findings provide insight into the molecular mechanisms underlying negative regulation of noncanonical TGF-β pathways. Transforming growth factor-β (TGF-β) family is a multifunctional cytokine involved in various cellular functions such as proliferation, apoptosis, differentiation and adult tissue homoeostasis [1] , [2] , [3] . A number of studies indicate that TGF-β signalling can be classified into two types of pathways depending on the availability of receptor-activated Smads (R-Smads): the Smad-dependent canonical pathway and Smad-independent noncanonical pathways. In the canonical pathway, TGF-β binding to type II (TβRII) and type I (TβRI) receptors initiates the signalling process through the intrinsic kinase activity of the receptors. Activated type I receptor transmits intracellular signals through phosphorylation of the R-Smads, Smad2 and Smad3. The phosphorylated R-Smads form heteromeric complexes with the Smad4 and translocate into the nucleus to modulate expression of diverse target genes [4] . Smad-independent noncanonical pathways include diverse intracellular signalling molecules such as TGF-β-associated kinase 1 (TAK1), p38 mitogen-activated protein kinase (p38 MAPK), c-Jun N-terminal kinase (JNK), extracellular signal regulated kinase (Erk), Rho-GTPase, and Akt [5] , [6] , [7] , [8] , [9] , [10] , [11] , [12] , [13] , but not the R-Smads. The TNF-receptor-associated factor 6 (TRAF6)-TAK1-p38 MAPK/JNK pathway is a well-characterized noncanonical TGF-β1 signalling pathway, where TRAF6 is crucial for TGF-β1-mediated activation of TAK1 (refs 14 , 15 , 16 ). TβRII/TβRI receptor complexes associate with TRAF6 upon binding to TGF-β1, inducing autoubiquitination of TRAF6 in a Lys63-dependent manner. Activated TRAF6 activates TAK1, presumably through ubiquitination and phosphorylation of TAK1, and results in the activation of downstream p38 MAPK/JNK [14] . The TGF-β signalling pathway needs to be carefully regulated to maintain tissue homoeostasis, because hyperactivation or hypoactivation of TGF-β signalling is highly related to human diseases including cancer [17] . Thus, much attention has been paid to the negative regulatory mechanisms of TGF-β signalling. Most works have focused on negative regulation of the Smad-dependent canonical TGF-β pathway to reveal that the inhibitory Smads (I-Smads), Smad7 and Smad6, act as antagonists of the canonical TGF-β pathway [18] , [19] , [20] . In particular, TGF-β1-induced Smad7 recruits Smad ubiquitin regulatory factor (Smurf) proteins with HECT type E3 ubiquitin ligase activity to suppress the canonical TGF-β pathway through ubiquitination-mediated proteasomal degradation of TβRI [21] , [22] . The role of Smad6 in the canonical TGF-β pathway has not been studied as much as Smad7 since Smad6 has been mainly recognized as a major antagonist of bone morphogenic protein (BMP) signalling that induces the degradation of R-Smads via recruitment of Smurfs [23] . Accumulating evidence indicates that Smad6 is also induced by TGF-β1 and may have additional roles in TGF-β signal transduction, such as being a mediator of the anti-inflammatory TGF-β signal [24] , [25] , [26] , [27] . Moreover, I-Smads can recruit specific deubiquitinating enzymes (DUBs) as well as E3 ubiquitin ligases [28] , [29] , suggesting that post-translational ubiquitination and deubiquitination of specific target proteins by I-Smads are important in regulation of the TGF-β signalling pathway. In contrast to the canonical TGF-β pathway, it is unknown how the noncanonical TGF-β-mediated pathway is negatively regulated. We here investigate whether the inhibitory Smads, Smad6 and Smad7, are involved in negative regulation of a noncanonical pathway. In particular, we provide in vitro and in vivo experimental evidence that Smad6 acts as a critical mediator that recruits the deubiquitinating enzyme A20 and inhibits TGF-β1-induced K63-linked polyubiquitination of TRAF6, contributing to negative regulation of the noncanonical TGF-β1-TRAF6-TAK1-p38 MAPK/JNK pathway. SMAD6 knockdown maintains TRAF6 polyubiquitination by TGF-β1 Since the inhibitory Smads, Smad6 and Smad7, are known as intrinsic antagonists of Smad-dependent canonical TGF-β/BMP signalling [18] , [20] , we questioned whether these proteins are involved in the negative regulation of TGF-β1-induced TRAF6-TAK1-p38 MAPK/JNK activation. We generated SMAD6 or SMAD7 knockdown AML-12 mouse liver cells, by infection of lentiviruses expressing one of two independent SMAD6 - or SMAD7 -specific small hairpin RNAs (shRNAs) ( Supplementary Fig. S1 ). TGF-β1-activated TAK1-p38/JNK signalling has been well studied in AML-12 mouse liver cells [15] . TGF-β1-induced endogenous TRAF6 polyubiquitination and downstream activation of TAK1 and p38/JNK was observed in the knockdown cells ( Fig. 1a ; Supplementary Fig. S2 ). Green fluorescent protein (GFP)-specific shRNA (shGFP) was used as a negative control. To exclude nonspecific binding to ubiquitin, cell lysates were boiled in lysis buffer containing 1% SDS and membrane filters containing SDS-PAGE-separated immunoprecipitates were treated with denaturation buffer containing 6 M guanidine chloride. TRAF6 was polyubiquitinated within 30 min, and polyubiquitination was promptly abolished after 1 h in TGF-β1-treated SMAD7 knockdown and shGFP-expressing control AML-12 cells ( Fig. 1a and Supplementary Fig. S2 ). Phosphorylation of downstream TAK1, p38 MAPK, and JNK was decreased in SMAD 7 knockdown cells compared to control cells, indicating that Smad7 is required for TGF-β1-induced activation of TAK1-p38 MAPK/JNK, consistent with a previous report [30] ; ( Fig. 1a and Supplementary Fig. S2 ). Smad6 expression was also transiently induced by TGF-β1 and inversely correlated with endogenous TRAF6 polyubiquitination and TAK1 and p38 MAPK/JNK phosphorylation in shGFP-expressing control AML-12 cells ( Fig. 1a ; Supplementary Fig. S2 ). Interestingly, TRAF6 ubiquitination was persistently activated up to 2 h in TGF-β1-treated SMAD6 knockdown AML-12 cells, compared to SMAD7 knockdown cells, and subsequent phosphorylation levels of TAK1and p38/JNK were maintained ( Fig. 1a ; Supplementary Fig. S2 ). Similar results were observed in SMAD6 -knockdown primary mouse hepatocytes ( Fig. 1b ), although the time points showing maximum polyubiquitination of TRAF6 in AML-12 and primary hepatocytes was different. The reason is likely to be due to differences in cell context between cell lines and primary cells. However, SMAD6 knockdown AML-12 cells or primary hepatocytes failed to inhibit Smad2 phosphorylation and expression of a Smad-specific (CAGA) reporter gene ( Fig. 1a–c ; Supplementary Fig. S2 ), compared to SMAD7 knockdown cells. These results indicate that Smad6 is involved in negative regulation of the TGF-β1-induced TRAF6-TAK1 noncanonical pathway through regulating TRAF6 polyubiquitination, but is not involved in negative regulation of the Smad-dependent canonical pathway. 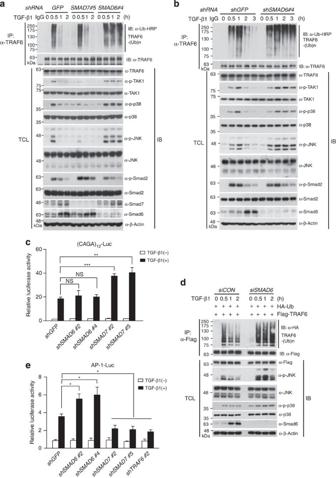Figure 1:SMAD6knockdown maintains TGF-β1-induced TRAF6 polyubiquitination. (a) AML-12 cells were infected with lentiviruses expressing shRNAs targetingSMAD6 orSMAD7, and treated with 5 ng ml−1TGF-β1 for the indicated times. Green fluorescence protein (GFP)-specific shRNA (shGFP) was used as a negative control. Endogenous TRAF6 ubiquitination was observed by immunoprecipitation (IP) with anti-TRAF6 antibody under denaturing conditions and immunoblotting (IB) with anti-ubiquitin-HRP. Total cell lysates (TCL) were immunoblotted by the indicated antibodies. (b) Mouse primary hepatocytes were infected with lentiviruses expressing shRNAs againstGFPorSMAD6, and treated with 5 ng ml−1TGF-β1 for the indicated times. Endogenous TRAF6 ubiquitination and phospho/total levels of TAK1, p38 MAPK, JNK, Smad2, and Smad6 were analysed by IB. (c) TGF-β1-induced transcriptional response inSMAD6orSMAD7knockdown AML-12 cells. Cells were transfected with a 12XCAGA-Luc reporter plasmid. After 24 h, cells were treated with TGF-β1 for 12 h, and luciferase activities were measured and normalized. (d)SMAD6knockdown CMT-93 cells were transfected with Flag-TRAF6 and HA-Ub plasmids, and treated with TGF-β1 for the indicated times. Flag-TRAF6 ubiquitination was examined by IP using anti-Flag antibody and subsequent IB with anti-HA. (e) AP-1-mediated transcriptional response inSMAD6orSMAD7knockdown AML-12 cells in the presence of TGF-β1. Cells were transfected with an AP-1-Luc reporter plasmid. After 24 h, cells were treated with TGF-β1 for 12 h, and luciferase activities were measured and normalized. The data in (c) and (e) are means ± s.d. (*P<0.05, **P<0.01, ***P<0.001,t-test;n=3). Expression of β-actin was used as a loading control in (a,b), and (d). All data are representative of at least three independent experiments. Figure 1: SMAD6 knockdown maintains TGF-β1-induced TRAF6 polyubiquitination. ( a ) AML-12 cells were infected with lentiviruses expressing shRNAs targeting SMAD 6 or SMAD7 , and treated with 5 ng ml −1 TGF-β1 for the indicated times. Green fluorescence protein (GFP)-specific shRNA (shGFP) was used as a negative control. Endogenous TRAF6 ubiquitination was observed by immunoprecipitation (IP) with anti-TRAF6 antibody under denaturing conditions and immunoblotting (IB) with anti-ubiquitin-HRP. Total cell lysates (TCL) were immunoblotted by the indicated antibodies. ( b ) Mouse primary hepatocytes were infected with lentiviruses expressing shRNAs against GFP or SMAD6 , and treated with 5 ng ml −1 TGF-β1 for the indicated times. Endogenous TRAF6 ubiquitination and phospho/total levels of TAK1, p38 MAPK, JNK, Smad2, and Smad6 were analysed by IB. ( c ) TGF-β1-induced transcriptional response in SMAD6 or SMAD7 knockdown AML-12 cells. Cells were transfected with a 12XCAGA-Luc reporter plasmid. After 24 h, cells were treated with TGF-β1 for 12 h, and luciferase activities were measured and normalized. ( d ) SMAD6 knockdown CMT-93 cells were transfected with Flag-TRAF6 and HA-Ub plasmids, and treated with TGF-β1 for the indicated times. Flag-TRAF6 ubiquitination was examined by IP using anti-Flag antibody and subsequent IB with anti-HA. ( e ) AP-1-mediated transcriptional response in SMAD6 or SMAD7 knockdown AML-12 cells in the presence of TGF-β1. Cells were transfected with an AP-1-Luc reporter plasmid. After 24 h, cells were treated with TGF-β1 for 12 h, and luciferase activities were measured and normalized. The data in ( c ) and ( e ) are means ± s.d. (* P <0.05, ** P <0.01, *** P <0.001, t -test; n =3). Expression of β-actin was used as a loading control in ( a , b ), and ( d ). All data are representative of at least three independent experiments. Full size image To test whether Smad6 is important for the negative regulation of TGF-β1-induced TRAF6 polyubiquitination at later time points, endogenous TRAF6 polyubiquitination was examined in SMAD6 knockdown or control AML-12 cells up until 8 h after TGF-β1 treatment. Decreased TRAF6 polyubiquitination was initially observed 1 h after TGF-β1 treatment and maintained at a decreased level up until 8 h in shGFP-expressing AML-12 cells ( Fig. 1a ; Supplementary Fig. S3a ). In contrast, Smad6 expression was significantly sustained from 1 h to 8 h in shGFP-expressing AML-12 cells ( Fig. 1a ; Supplementary Fig. S3a ). Interestingly, polyubiquitinated TRAF6 persisted until 4 h after TGF-β1 treatment, and gradually decreased in SMAD6 knockdown cells at 8 h ( Supplementary Fig. S3a ). Also, the subsequent phosphorylation of downstream TAK1 was similar to the patterns of TRAF6 ubiquitination in SMAD6 knockdown cells ( Supplementary Fig. S3a ). The sustained ubiquitination of TRAF6 in SMAD6 knockdown AML-12 cells was completely abolished in a shSMAD6#4-resistant silent mutant Flag-Smad6 ( Supplementary Fig. S3b ; Supplementary Table S1 ). Immunoprecipitation and ubiquitination assays of ectopically expressed TRAF6 in SMAD6 knockdown CMT-93 mouse epithelial cells support these conclusions ( Fig. 1d ). Since p38 MAPK/JNK activate the activator protein-1 (AP-1) transcription factor which consists of c-Jun and c-Fos, we next examined whether TGF-β1 increases AP-1 activity in SMAD6 knock-down cells. The activity of a AP-1-mediated reporter was significantly increased in SMAD6 knockdown AML-12 cells, and decreased in both SMAD7 knockdown and TRAF6 knockdown (shTRAF6) AML-12 cells which were used as a control ( Fig. 1e ; Supplementary Fig. S4a ). Smad6 inhibits TRAF6 polyubiquitination TRAF6 is autoubiquitinated in TGF-β1-induced TRAF6 activation [14] , [15] . To verify the inhibitory effects of Smad6 on TRAF6 polyubiquitination, plasmids encoding His-tagged ubiquitin, Flag-TRAF6, HA-SMAD6 or HA-SMAD7 were transiently transfected into HEK293 human embryonic kidney cells as indicated ( Fig. 2a,b,d ). TRAF6 polyubiquitination was examined under denaturing conditions of 6 M guanidine-HCl by a Ni-NTA agarose-mediated pull-down experiment. As expected, Smad6 inhibited TRAF6 polyubiquitination in a dose-dependent manner ( Fig. 2a ). To identify which polyubiquitination patterns of TRAF6 are affected by Smad6, wild-type ubiquitin, the K48 ubiquitin mutant in which six lysine residues except for lysine 48 are substituted into arginines, and the K63 mutant in which only lysine 63 is left intact, were transfected into HEK293 cells with Flag-TRAF6 in the absence or presence of HA-Smad6. Smad6 specifically inhibited K63-linked polyubiquitination of TRAF6, but not K48-linked one ( Fig. 2b ). Immunoblot analysis using an antibody against K63-specific ubiquitin (Ub)-horseradish peroxidase (HRP) supported our results that Smad6 inhibits K63-linked polyubiquitination on endogenous TRAF6 in AML-12 cells ( Fig. 2c ). Furthermore, an Ni-NTA agarose-mediated pull-down assay indicated that Smad7 does not inhibit TRAF6 polyubiquitination and that the inhibitory effects of Smad6 on TRAF6 are similar to the A20 deubiquitinating enzyme [31] , [32] ; ( Fig. 2d ). Next, we investigated whether Smad6 regulates TAK1 polyubiquitination in the overexpression system in HEK293 cell. TAK1 is a downstream effector of TRAF6 whose polyubiquitination is crucial for activation [33] , [34] . Smad6 did not directly inhibit polyubiquitination of TAK1 protein under these conditions ( Fig. 2e ), compared to TRAF6. This may be because HEK293 cells, which do not show significant responsiveness to TGF-β1, were not treated with TGF-β1, or because Smad6 may be indirectly involved in TAK1 deubiquitination through TRAF6 deubiquitination in the presence of TGF-β1. Therefore, to verify whether Smad6 is indirectly involved in the deubiquitination of TGF-β1-induced TAK1 polyubiquitination, we examined the ubiquitination of endogenous TAK1 protein in SMAD6 knockdown AML-12 cells upon TGF-β1 treatment. Ubiquitination of the TAK1 protein was maximal at 30 min after TGF-β1 treatment and subsequently decreased in shGFP-expressing AML-12 cells, whereas they persisted in SMAD6 knockdown AML-12 cells ( Fig. 2f ). Together with the results of TAK1 polyubiquitintaion by Smad6 in HEK293 cells ( Fig. 2e ), this sustained ubiquitination of endogenous TAK1 in SMAD6 knockdown cells in the presence of TGF-β1 is likely due to persistant ubiquitination of TRAF6 by knockdown of the SMAD6 gene. Collectively, our present findings suggest that Smad6 specifically inhibits TRAF6 polyubiquitination but not directly TAK1, in the TGF-β1-induced TRAF6-TAK1 noncanonical pathway. 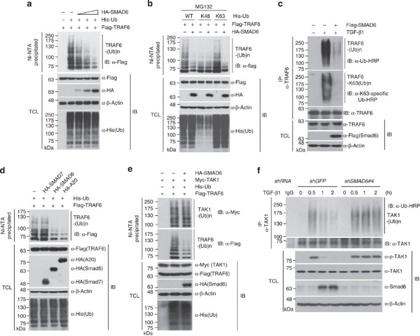Figure 2: Smad6 downregulates TRAF6 polyubiquitination. (a) Smad6 inhibits TRAF6 polyubiquitination in a dose-dependent manner. Plasmids encoding Flag-TRAF6 and His-Ub were co-transfected with increasing amounts of HA-SMAD6 plasmid into HEK293 cells. (b) Plasmids encoding wild-type or lysine mutants (K48 and K63) of His-Ub were co-transfected with Flag-TRAF6 and HA-SMAD6 plasmids into HEK293 cells. Cells were treated with the proteasome inhibitor MG132 for 4 h, and Ni-NTA-mediated pull-down assays were performed. (c) Plasmid encoding Flag-SMAD6 was transfected into AML-12 cells and treated with TGF-β1 for 30 min. After IP against endogenous TRAF6, K63-linked polyubiquitination of TRAF6 was observed by IB using a K63-specific ubiquitin antibody. (d) Plasmids encoding Flag-TRAF6 and His-Ub were co-transfected with HA-SMAD6, HA-SMAD7, and HA-A20 plasmids, respectively. (e) Smad6 specifically inhibits TRAF6 ubiquitination, but not TAK1. Plasmids encoding Flag-TRAF6, Myc-TAK1, His-Ub, and HA-SMAD6 were co-transfected into HEK293 cells in the indicated combinations. The ubiquitinated proteins and total cell lysates were observed by Ni-NTA-mediated pull-down assay and IB using the indicated antibodies. (f) AML-12 cells were infected with lentiviruses expressing shRNAs targeting GFP (shGFP; negative control ) or shSMAD6#4 and treated with 5 ng ml−1TGF-β1 for the indicated times. Endogenous TAK1 ubiquitination was observed by immunoprecipitation under denaturing conditions with an anti-TAK1 antibody and immunoblotted with anti-ubiquitin-HRP. Total cell lysates were immunoblotted with indicated antibodies. Expression of the β-actin was used as a loading control. All data are representative of at least three independent experiments. Figure 2: Smad6 downregulates TRAF6 polyubiquitination. ( a ) Smad6 inhibits TRAF6 polyubiquitination in a dose-dependent manner. Plasmids encoding Flag-TRAF6 and His-Ub were co-transfected with increasing amounts of HA-SMAD6 plasmid into HEK293 cells. ( b ) Plasmids encoding wild-type or lysine mutants (K48 and K63) of His-Ub were co-transfected with Flag-TRAF6 and HA-SMAD6 plasmids into HEK293 cells. Cells were treated with the proteasome inhibitor MG132 for 4 h, and Ni-NTA-mediated pull-down assays were performed. ( c ) Plasmid encoding Flag-SMAD6 was transfected into AML-12 cells and treated with TGF-β1 for 30 min. After IP against endogenous TRAF6, K63-linked polyubiquitination of TRAF6 was observed by IB using a K63-specific ubiquitin antibody. ( d ) Plasmids encoding Flag-TRAF6 and His-Ub were co-transfected with HA-SMAD6, HA-SMAD7, and HA-A20 plasmids, respectively. ( e ) Smad6 specifically inhibits TRAF6 ubiquitination, but not TAK1. Plasmids encoding Flag-TRAF6, Myc-TAK1, His-Ub, and HA-SMAD6 were co-transfected into HEK293 cells in the indicated combinations. The ubiquitinated proteins and total cell lysates were observed by Ni-NTA-mediated pull-down assay and IB using the indicated antibodies. ( f ) AML-12 cells were infected with lentiviruses expressing shRNAs targeting GFP (shGFP; negative control ) or shSMAD6#4 and treated with 5 ng ml −1 TGF-β1 for the indicated times. Endogenous TAK1 ubiquitination was observed by immunoprecipitation under denaturing conditions with an anti-TAK1 antibody and immunoblotted with anti-ubiquitin-HRP. Total cell lysates were immunoblotted with indicated antibodies. Expression of the β-actin was used as a loading control. All data are representative of at least three independent experiments. Full size image A20 suppresses TGF-β1-mediated TAK1-p38 MAPK/JNK activation We hypothesized that Smad6 recruits a specific deubiquitinating enzyme (DUB) to deubiquitinate TRAF6, since Smad6 does not have a domain with deubiquitinating activity. Since the DUBs A20 and cylindromatosis tumour suppressor (CYLD) negatively regulate lipopolysaccharide/interlukin-1β (LPS/IL-1β) or tumour necrosis factor-α (TNF-α)- induced NF-κB signalling by deubiquitinating TRAF6/RIP1 (refs 31 , 32 , 35 ), we examined whether A20 or CYLD is involved in Smad6-mediated TRAF6 deubiquitination. First, plasmids encoding HA-SMAD6, His-ubiquitin, and Flag-TRAF6 were transfected into HEK293 cells expressing A20 - or CYLD -specific siRNAs ( Supplementary Fig. S4b ). As a control, plasmids were transfected into HEK293 cells expressing scrambled siRNAs (siCON). Ni-NTA agarose pull-down assays indicated that deubiquitination of polyubiqutinated TRAF6 in the presence of Smad6 was suppressed in A20 knockdown cells, but not in CYLD knockdown cells ( Fig. 3a ). We next examined whether A20 deubiquitinates endogenous TRAF6 upon TGF-β1 treatment and subsequently inhibits phosphorylation of the downstream TAK1 and p38 MAPK/JNK in AML-12 cells ( Fig. 3b ). Similar to SMAD6 knockdown AML-12 cells, TRAF6 polyubiquitination persisted in different shRNA-expressing A20 knockdown AML-12 cells, but was not observed in CYLD knockdown cells ( Fig. 3b,c ; Supplementary Fig. S4c ). In addition, TAK1 and p38 MAPK/JNK phosphorylation was maintained only in A20 knockdown AML-12 cells ( Fig. 3b,c ). Interestingly, Smad2 phosphorylation was decreased in A20 knockdown cells but not affected in SMAD6 knockdown AML-12 cells, indicating that A20 plays a role in the canonical TGF-β pathway as well as noncanonical pathway. Consistent results regarding the function of A20 in TGF-β1-induced TRAF6-TAK1-p38 MAPK/JNK activation were obtained in A20 knockdown primary hepatocytes ( Fig. 3d ). The expression level of endogenous A20 in AML-12 mouse liver cells and primary hepatocytes was relatively higher than bone marrow-derived macrophages (BMDM), suggesting that endogenous A20 levels are likely to be dependent on cell types ( Supplementary Fig. S5 ). 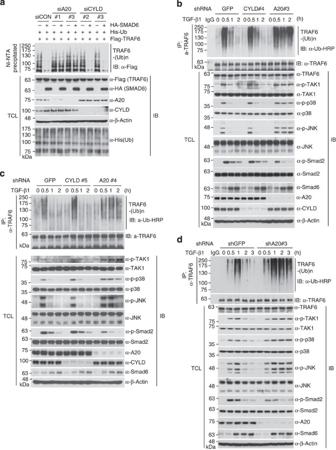Figure 3: Knockdown ofA20sustains TGF-β1-mediated TRAF6 polyubiquitination. (a) A20, but not CYLD, is required for Smad6-mediated inhibition of TRAF6 polyubiquitination. HEK293 cells were reverse-transfected with 30 nM of control siRNA (siCON) or two independent A20 siRNAs (siA20#1 or #3) or CYLD siRNAs (siCYLD #2 or #3), respectively. After 24 h, Flag-TRAF6 and His-Ub plasmids were co-transfected with HA-SMAD6 into HEK293 cells in the indicated combinations. Cells were lysed in 6 M guanidine-HCl, and His-ubiquitinated proteins precipitated using Ni-NTA agarose beads. Ubiquitinated TRAF6 was observed by IB using anti-Flag antibody. (b–d) AML-12 cells (b,c) and mouse primary hepatocytes (d) were infected with lentiviruses expressing the indicated shRNAs targetingGFP(shGFP; negative control ),A20, orCYLD, and treated with 5 ng ml−1TGF-β1 for the indicated times. For (b–d), endogenous TRAF6 ubiquitination was observed by IP under denaturing conditions with anti-TRAF6 antibody and immunoblotted with anti-ubiquitin-HRP. Total cell lysates were immunoblotted with indicated antibodies. Expression of β-actin was used as a loading control. The data in (a–d) are representative of at least three independent experiments. Figure 3: Knockdown of A20 sustains TGF-β1-mediated TRAF6 polyubiquitination. ( a ) A20, but not CYLD, is required for Smad6-mediated inhibition of TRAF6 polyubiquitination. HEK293 cells were reverse-transfected with 30 nM of control siRNA (siCON) or two independent A20 siRNAs (siA20#1 or #3) or CYLD siRNAs (siCYLD #2 or #3), respectively. After 24 h, Flag-TRAF6 and His-Ub plasmids were co-transfected with HA-SMAD6 into HEK293 cells in the indicated combinations. Cells were lysed in 6 M guanidine-HCl, and His-ubiquitinated proteins precipitated using Ni-NTA agarose beads. Ubiquitinated TRAF6 was observed by IB using anti-Flag antibody. ( b – d ) AML-12 cells ( b , c ) and mouse primary hepatocytes ( d ) were infected with lentiviruses expressing the indicated shRNAs targeting GFP (shGFP; negative control ), A20 , or CYLD , and treated with 5 ng ml −1 TGF-β1 for the indicated times. For ( b – d ), endogenous TRAF6 ubiquitination was observed by IP under denaturing conditions with anti-TRAF6 antibody and immunoblotted with anti-ubiquitin-HRP. Total cell lysates were immunoblotted with indicated antibodies. Expression of β-actin was used as a loading control. The data in ( a – d ) are representative of at least three independent experiments. Full size image Similar to SMAD6 knockdown AML-12 cells at later time points, the deubiquitination of TRAF6 persisted until 4 h after TGF-β1 treatment, and gradually decreased in A20 knockdown cells at 8 h ( Supplementary Fig. S6a ). Also subsequent phosphorylation patterns of downstream TAK1 were similar to TRAF6 ubqiuitination patterns ( Supplementary Fig. S6a ). Sustained TRAF6 ubiquitination in A20 knockdown AML-12 cells was completely abolished in shA20#3-resistant human Flag-A20 protein transfected cells ( Supplementary Fig. S6b ). To verify that A20 is involved in the regulation of TGF-β1-induced TRAF6 polyubiquitination, plasmids encoding an A20 wild-type gene or A20 ( C103A ) mutant with the catalytic cysteine residue showing DUB activity substituted into alanine were transfected into AML-12 cells, and the cells were treated with TGF-β1 for 30 min. Although wild type A20 and its mutant A20(C103A) proteins bound to endogenous TRAF6 and Smad6 ( Fig. 4a ), wild-type A20 inhibited endogenous TRAF6 polyubiquitination whereas mutant A20(C103A) failed to deubiquitinate TRAF6 ( Fig. 4b , lane 3,4), providing support that the catalytic activity of A20 is required for deubiquitination of TGF-β1-induced TRAF6 polyubiquitination. To further confirm this, we generated two zinc finger (ZF) mutants, in which the tyrosine and phenylalanine residues of ZF4 and the phenylalanine and glycine residues of ZF7 were substituted into alanines, as previously described [36] , [37] . The non-enzymatic ZF4 and ZF7 domains are known to bind to K63-linked polyubiquitin chains and inhibit NF-κB signalling [36] , [37] , although recent results regarding ZF7, emphasize that ZF7 mainly binds to linear polyubiquitin chains [38] , [39] . The ZF4 and ZF7 mutants bound to TRAF6 ( Fig. 4c ). However, the ZF7 mutant still inhibited endogenous TRAF6 deubiquitination as much as wild-type A20, demonstrating that the ZF7 domain is not involved in A20-mediated deubiquitination of TRAF6 in the presence of TGF-β1 ( Fig. 4b , lane 6 and Fig. 4d ). Interestingly, the ZF4 mutant partially affected the deubiquitination of TRAF6 ( Fig. 4b , lane 5, and Fig. 4d ). These results indicate that the enzymatic deubiquitinase activity of A20 is mainly involved in the deubiquitination of TGF-β1-induced TRAF6 ubiquitination and the ZF4 domain is partly involved in negative regulation of TRAF6 ubiquitination in the presence of TGF-β1. 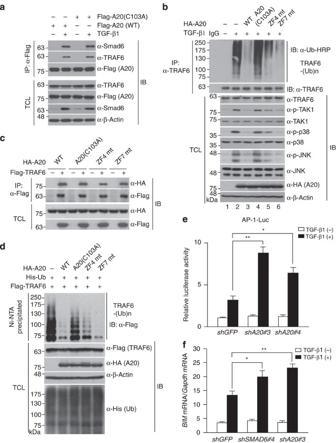Figure 4: Interaction of A20 mutants with TRAF6 and their deubiquitinating activity. (a) Plasmids encoding a catalytic inactive mutant (A20(C103A)) or wild-type A20 were transfected into AML-12 cells in the indicated combinations and subsequently treated with TGF-β1 for 2 h. After immunoprecipitation (IP) with anti-Flag antibody, the interaction of endogenous Smad6 and TRAF6 with wild-type A20 or A20 mutant A20(C103A) was detected by immunoblotting (IB). (b) Plasmids expressing wild-type A20, a catalytically inactive DUB mutant of A20(C103A), ZF4 mutant (Y614A/F615A), or ZF7 mutant (F770A/G771A) were transfected into AML-12 cells and treated with 5 ng ml−1TGF-β1 for 30 min. For (b–d), endogenous TRAF6 ubiquitination was observed by IP under denaturing conditions with anti-TRAF6 antibody and immunoblotted with anti-ubiquitin-HRP. (c) Plasmids encoding a catalytic inactive mutant (A20(C103A)), ZF4 mutant (ZF4 mt; Y614A/F615A), or ZF7 mutant (ZF7 mt; F770A/G771A) were transiently co-transfected with wild-type Flag-TRAF6 into HEK293 cells. IP and IB were performed with the indicated antibodies. (d) The A20 mutants were co-transfected with plasmids encoding His-Ub and Flag-TRAF6 into HEK293 cells in the indicated combinations. And Ni-NTA-mediated pull-down assays were performed. For (a–d), total cell lysates were immunoblotted with indicated antibodies. Expression of β-actin was used as a loading control. The data in (a–d) are representative of at least three independent experiments. (e) AP-1-mediated reporter activity inA20knockdown AML-12 cells upon TGF-β1 treatment. Cells were transfected with AP-1-Luc. After 24 h, cells were treated with TGF-β1 for 12 h and luciferase activity was measured and normalized. (f) Expression ofBIMmRNA was analysed by quantitative real-time RT-PCR inA20orSMAD6knockdown AML-12 cells treated with TGF-β1 for 1 h. The data are means ± s.d. (*P<0.05, **P<0.01,t-test;n=3). Figure 4: Interaction of A20 mutants with TRAF6 and their deubiquitinating activity. ( a ) Plasmids encoding a catalytic inactive mutant (A20(C103A)) or wild-type A20 were transfected into AML-12 cells in the indicated combinations and subsequently treated with TGF-β1 for 2 h. After immunoprecipitation (IP) with anti-Flag antibody, the interaction of endogenous Smad6 and TRAF6 with wild-type A20 or A20 mutant A20(C103A) was detected by immunoblotting (IB). ( b ) Plasmids expressing wild-type A20, a catalytically inactive DUB mutant of A20(C103A), ZF4 mutant (Y614A/F615A), or ZF7 mutant (F770A/G771A) were transfected into AML-12 cells and treated with 5 ng ml −1 TGF-β1 for 30 min. For ( b – d ), endogenous TRAF6 ubiquitination was observed by IP under denaturing conditions with anti-TRAF6 antibody and immunoblotted with anti-ubiquitin-HRP. ( c ) Plasmids encoding a catalytic inactive mutant (A20(C103A)), ZF4 mutant (ZF4 mt; Y614A/F615A), or ZF7 mutant (ZF7 mt; F770A/G771A) were transiently co-transfected with wild-type Flag-TRAF6 into HEK293 cells. IP and IB were performed with the indicated antibodies. ( d ) The A20 mutants were co-transfected with plasmids encoding His-Ub and Flag-TRAF6 into HEK293 cells in the indicated combinations. And Ni-NTA-mediated pull-down assays were performed. For ( a – d ), total cell lysates were immunoblotted with indicated antibodies. Expression of β-actin was used as a loading control. The data in ( a – d ) are representative of at least three independent experiments. ( e ) AP-1-mediated reporter activity in A20 knockdown AML-12 cells upon TGF-β1 treatment. Cells were transfected with AP-1-Luc. After 24 h, cells were treated with TGF-β1 for 12 h and luciferase activity was measured and normalized. ( f ) Expression of BIM mRNA was analysed by quantitative real-time RT-PCR in A20 or SMAD6 knockdown AML-12 cells treated with TGF-β1 for 1 h. The data are means ± s.d. (* P <0.05, ** P <0.01, t -test; n =3). Full size image Also, the findings that A20 knockdown sustains TRAF6 polyubiquitination prompted us to investigate AP-1 activity, which is a downstream target of p38 MAPK/JNK. AP-1 reporter activity was increased in A20 knockdown AML-12 cells upon TGF-β1 treatment compared to shGFP-expressing control cells ( Fig. 4e ). Furthermore, quantitative real-time RT-PCR analysis of the pro-apoptotic BIM gene, which is one of target genes controlled by AP-1 (ref. 40 ), showed that BIM mRNAs are significantly increased in SMAD6 or A20 knockdown AML-12 cells upon TGF-β1 treatment, supporting our results ( Fig. 4f ). Therefore, our findings suggest that the A20 protein is required for the deubiquitination of TGF-β1-induced TRAF6 polyubiquitination, leading to downregulation of TAK1-p38/JNK activation. A20-meidated deubiquitination of TRAF6 requires Smad6 Next we examined whether Smad6 is required for A20-mediated deubiquitination of TRAF6 in TGF-β1-induced TRAF6-TAK1 activation. A plasmid encoding Flag-A20 was transfected into SMAD6 knockdown or shGFP-expressing control AML-12 cells. After TGF-β1 treatment for 45 min, ubiquitination assays for endogenous TRAF6 were performed ( Fig. 5a ). Ectopic expression of Flag-A20 significantly inhibited the polyubiquitination of TRAF6 in control AML-12 cells (lane 3) but not in SMAD6 knockdown AML-12 cells (lane 6), indicating that Smad6 is required for A20-mediated deubiquitination of TRAF6 ( Fig. 5a ). 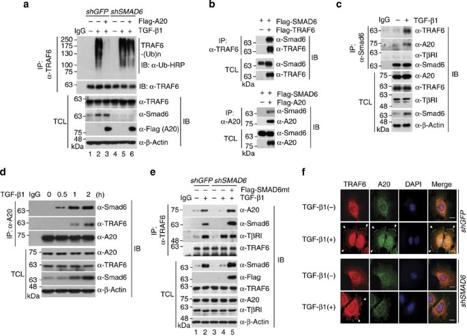Figure 5: Smad6 recruits A20 to polyubiquitinated TRAF6 in response to TGF-β1. (a) AML-12 cells were infected with lentiviruses expressing shRNAs targeting GFP (negative control) orSMAD6and subsequently transfected with a plasmid encoding Flag-A20. Upon TGF-β1 treatment for 45 min, endogenous TRAF6 ubiquitination was observed by IP with anti-TRAF6 antibody under denaturing conditions and IB with anti-ubiquitin-HRP. (b) Plasmids encoding Flag-SMAD6 was co-transfected with Flag-TRAF6 or Flag-A20 into HEK293 cells. Cell lysates were immunoprecipitated with indicated antibodies and analysed by IB. (c) Interactions between Smad6, TRAF6 and A20. AML-12 cells were treated with TGF-β1 for 2 h. To confirm the interaction of endogenous Smad6, TRAF6, and A20 proteins, IP and IB were performed with the indicated antibodies against endogenous proteins. (d) Time-dependent formation of endogenous trimeric Smad6-TRAF6-A20 complex was monitored by IP and IB upon TGF-β1 treatment in AML-12 cells. (e) Re-expression of an shRNA-resistant silent mutantSMAD6gene inSMAD6knockdown AML-12 cells restores the interaction between TRAF6 and A20. IP and IB were performed with the indicated antibodies. (f)SMAD6knockdown reduces the recruitment of A20 to TRAF6 at the plasma membrane in the presence of TGF-β1. Immunofluorescence and DAPI staining of TRAF6 and A20 inSMAD6knockdown or control AML-12 cells. Cells were treated with TGF-β1 for 2 h. Arrow heads indicate plasma-membrane localization. Scale bar, 10 μm. Figure 5: Smad6 recruits A20 to polyubiquitinated TRAF6 in response to TGF-β1. ( a ) AML-12 cells were infected with lentiviruses expressing shRNAs targeting GFP (negative control) or SMAD6 and subsequently transfected with a plasmid encoding Flag-A20. Upon TGF-β1 treatment for 45 min, endogenous TRAF6 ubiquitination was observed by IP with anti-TRAF6 antibody under denaturing conditions and IB with anti-ubiquitin-HRP. ( b ) Plasmids encoding Flag-SMAD6 was co-transfected with Flag-TRAF6 or Flag-A20 into HEK293 cells. Cell lysates were immunoprecipitated with indicated antibodies and analysed by IB. ( c ) Interactions between Smad6, TRAF6 and A20. AML-12 cells were treated with TGF-β1 for 2 h. To confirm the interaction of endogenous Smad6, TRAF6, and A20 proteins, IP and IB were performed with the indicated antibodies against endogenous proteins. ( d ) Time-dependent formation of endogenous trimeric Smad6-TRAF6-A20 complex was monitored by IP and IB upon TGF-β1 treatment in AML-12 cells. ( e ) Re-expression of an shRNA-resistant silent mutant SMAD6 gene in SMAD6 knockdown AML-12 cells restores the interaction between TRAF6 and A20. IP and IB were performed with the indicated antibodies. ( f ) SMAD6 knockdown reduces the recruitment of A20 to TRAF6 at the plasma membrane in the presence of TGF-β1. Immunofluorescence and DAPI staining of TRAF6 and A20 in SMAD6 knockdown or control AML-12 cells. Cells were treated with TGF-β1 for 2 h. Arrow heads indicate plasma-membrane localization. Scale bar, 10 μm. Full size image We next investigated how Smad6 interacts with the TRAF6 and A20 proteins in the TGF-β1-induced TRAF6-TAK1 noncanonical pathway. Interaction between TRAF6 and A20 has been previously reported [41] . Co-immunoprecipitation assays in overexpression systems indicated that Smad6 binds to the TRAF6 and A20 proteins, respectively ( Fig. 5b ). TGF-β1-induced endogenous Smad6 interacted with endogenous TRAF6 and A20 proteins in AML-12 cells and mouse primary hepatocytes ( Fig. 5c ; Supplementary Fig. S7a ). However, Smad6 did not bind to endogenous TβRI protein ( Fig. 5c ), although Smad6 has been reported to bind to TβRI in an overexpression system [20] , [42] . Formation of the endogenous trimeric complex, Smad6-A20-TRAF6 was maximized at 2 h after TGF-β1 treatment in AML-12 cells and at 3 h in primary hepatocytes ( Fig. 5d ; Supplementary Fig. S7b ). These were dependent on the maximal induction of Smad6 expression ( Fig. 5d ; Supplementary Fig. S7b ). The formation of the trimeric complex at 2 h or 3 h is consistent with the results showing maximum deubiquitination of TRAF6 ( Fig. 1a,b ). Furthermore, immunoprecipitation assays against endogenous TRAF6 in shGFP or shSMAD6-expressing AML-12 cells clearly indicate that TGF-β1-induced interaction between TRAF6 and A20 is dependent on the presence of Smad6, whereas TRAF6 bound to TβRI upon TGF-β1 treatment regardless of the presence of Smad6 ( Fig. 5e , lane 2,4). The basal binding of TRAF6 to TβRI in the absence of TGF-β1 supported the previous findings [14] , [15] ; ( Fig. 5e , lane 1). As the binding of TRAF6 with TβRI has been reported to be crucial for TRAF6 polyubiquitination [14] , [15] , these results imply that Smad6 does not participate in the initial signalling by TβRI and TRAF6 in the noncanonical TGF-β pathway, but specifically mediates the binding of A20 to TRAF6. Consistently, ectopic expression of a shRNA-resistant silent mutant Smad6 in SMAD6 knockdown AML-12 cells restored their interactions ( Fig. 5e , lane 5). Next, to verify the role of Smad6 on recruitiment of A20 to TRAF6, we performed immunofluorescence assays to observe subcellular localization in SMAD6 knockdown and control AML-12 cells in the absence or presence of TGF-β1. As previously reported [14] , TRAF6 colocalized with TβRI in the plasma membrane of control AML-12 cells upon TGF-β1 treatment ( Supplementary Fig. S7c ). In addition, some A20 proteins colocalized with TRAF6 in the plasma membrane of control AML-12 cells in the presence of TGF-β1 ( Fig. 5f ). A20 failed to colocalize to the plasma membrane of SMAD6 knockdown AML-12 cells although TRAF6 was still localized at the plasma membrane ( Fig. 5f ), demonstrating that Smad6 is a component critical to recruiting A20 to TRAF6 at the plasma membrane in the presence of TGF-β1. Also, considerable amounts of A20 translocated into the nucleus upon TGF-β1 treatment ( Fig. 5f ), implying that A20 may have additional functions in TGF-β signalling. Subcellular fractionation experiments supported the results of the colocalization experiments ( Supplementary Fig. S7d ). In control AML-12 cells, A20 was observed in the membrane fraction (ME) with TRAF6 in the presence of TGF-β1 ( Supplementary Fig. S7d , lane 2), whereas A20 was not in the membrane fraction (ME) in SMAD6 knockdown AML-12 cells as much as the control cells ( Supplementary Fig. S7d , lane 8). Two independent immunoblot analysis of Smad6, according to exposure time, indicated that part of Smad6 is observed in the membrane fraction (ME) with A20 and TRAF6 in control AML-12 cells upon TGF-β1 treatment ( Supplementary Fig. S7d , lane 2). Interestingly, TAK1 proteins were significantly increased in the ME upon TGF-β1 treatment regardless of the presence of Smad6 ( Supplementary Fig. S7e , lane 2,8), although most TAK1 were localized in the cytoplasmic fraction. Therefore, the recruitment of A20 to TRAF6 through TGF-β1-induced Smad6 expression seems to be critical for negative regulation of TGF-β1-mediated TRAF6-TAK1 activation, but not the changes of cellular localization of TAK1. These results collectively demonstrate that Smad6 is a crucial factor to recruit A20 to TRAF6. Smad6 bind differentially to TRAF6 and A20 We next examined which domains of Smad6 participate in the interactions with TRAF6 and A20. Three truncated mutants of Smad6, MH1-like, Linker, and MH2 domain [26] ( Supplementary Fig. S8 ), were transfected into HEK293 cells with full-length TRAF6 (Flag-TRAF6) or full-length A20 (Flag-A20). Co-immunoprecipitation assays revealed that the MH2 domain (amino acids 332 to 496) of Smad6 binds to TRAF6 whereas the linker domain (amino acids 181 to 331) binds to A20 ( Fig. 6a,b ). 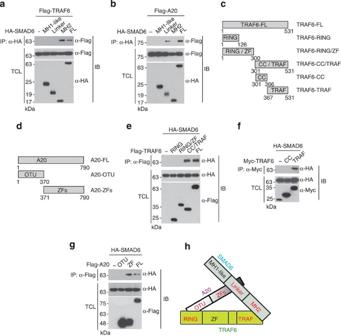Figure 6: Smad6 interacts with TRAF6 and A20 through different domains. (a,b) The Linker and MH2 regions of Smad6 interact with TRAF6 and A20, respectively. Truncated Smad6 mutants were co-transfected with the (a) full length Flag-TRAF6 plasmid or (b) full length Flag-A20 into HEK293 cells. IP and IB were performed with indicated antibodies. (c,d) Schematic representations of plasmids encoding different truncated forms of (c) TRAF6 and (d) A20. (e,f) Plasmids encoding truncated mutants of TRAF6 were co-transfected with full length HA-Smad6 plasmid into HEK293 cells. IP and IB were performed with the indicated antibodies. (g) Plasmids encoding truncated mutants of A20 were co-transfected with full length HA-Smad6 plasmid into HEK293 cells. IP and IB were performed with the indicated antibodies. (h) Schematic diagram of the interactions among Smad6, TRAF6, and A20. All data are representative of at least three independent experiments. Figure 6: Smad6 interacts with TRAF6 and A20 through different domains. ( a , b ) The Linker and MH2 regions of Smad6 interact with TRAF6 and A20, respectively. Truncated Smad6 mutants were co-transfected with the ( a ) full length Flag-TRAF6 plasmid or ( b ) full length Flag-A20 into HEK293 cells. IP and IB were performed with indicated antibodies. ( c , d ) Schematic representations of plasmids encoding different truncated forms of ( c ) TRAF6 and ( d ) A20. ( e , f ) Plasmids encoding truncated mutants of TRAF6 were co-transfected with full length HA-Smad6 plasmid into HEK293 cells. IP and IB were performed with the indicated antibodies. ( g ) Plasmids encoding truncated mutants of A20 were co-transfected with full length HA-Smad6 plasmid into HEK293 cells. IP and IB were performed with the indicated antibodies. ( h ) Schematic diagram of the interactions among Smad6, TRAF6, and A20. All data are representative of at least three independent experiments. Full size image To identify which domains of TRAF6 and A20 bind to Smad6, we generated five truncated mutants of TRAF6 (ref. 43 ); ( Fig. 6c ) and two truncated mutants of A20 ( Fig. 6d ). Co-immunoprecipitation assays indicated that the TRAF homology domain of TRAF6 (amino acids 367 to 531) is sufficient for binding with Smad6 ( Fig. 6e,f ) and the zinc finger (ZF) containing domain of A20 (amino acids 371 to 790) binds to Smad6 ( Fig. 6g ). Taking into consideration a previous finding that the OTU domain of A20 interacts with TRAF6 (ref. 44 ), these results demonstrate that distinct domains of Smad6 differentially interact with specific domains of TRAF6 and A20, forming Smad6-A20-TRAF6 complexes ( Fig. 6h ). Both Smad6 and A20 inhibit TGF-β-induced apoptosis Next, we examined the physiological roles of Smad6 and A20 in TGF-β1-induced TRAF6-TAK1 activation. Since the activation of TAK1-p38 MAPK/JNK signal has been closely linked to TGF-β1-mediated apoptosis [45] , [46] , we first investigated whether Smad6 and A20 are involved in TGF-β1-mediated apoptosis by Annexin-V staining and subG1 fraction analysis in SMAD6 knockdown and A20 knockdown AML-12 cells ( Fig. 7a–d ). In control AML-12 cells expressing shGFP, TGF-β1 treatment led to cellular apoptosis in serum-starved conditions ( Fig. 7a–d ). TGF-β1-mediated apoptosis was further increased in SMAD6 or A20 knockdown AML-12 cells ( Fig. 7a–d ). This can be attributed to sustained activation of the TRAF6-TAK1-p38 MAPK/JNK pathway upon inhibition of TRAF6 deubiquitination by SMAD6 or A20 knockdown. Consistent with these results, TRAF6 or SMAD7 knockdown reduced TGF-β1-mediated apoptotic cell death ( Fig. 7a–d ), indicating that the TGF-β1-TRAF6-TAK1 pathway is responsible for TGF-β1-mediated apoptosis in AML-12 cells and that Smad7 is a positive regulator in this apoptotic pathway. Detection of apoptotic markers such as PARP-1 and caspase-3 provided additional evidence that Smad6 and A20 are involved in negative regulation of TGF-β1-mediated apoptosis ( Fig. 7e ). Expression of cleaved PARP1 and caspase-3 was higher in SMAD6 or A20 knockdown AML-12 cells compared to control cells, and expression of PARP-1 and cleaved caspase-3 was further decreased in TRAF6 and SMAD7 knockdown AML-12 cells ( Fig. 7e,f ). 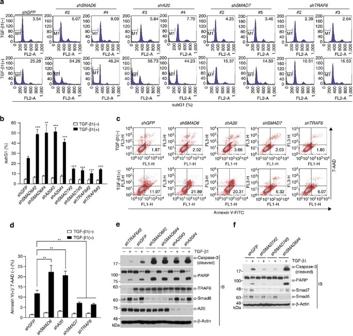Figure 7:SMAD6orA20knockdown enhances TGF-β1-induced apoptosis. (a–d) AML-12 cells were infected with lentiviruses expressing the indicated shRNAs and treated with TGF-β1 for 36 h under serum-starved conditions. (a) Cells were stained with propidium iodide (PI) and analysed by flow cytometry The percentages of the subG1 fraction are indicated. (b) The percentages of the subG1 fraction are summarized in a bar graph. The data are means ± s.d. (**P<0.01, ***P<0.001 compared with ‘shGFP with TGF-β1(+)’,t-test;n=3). (c) Cells were immediately stained with Annexin V and 7-AAD, and analysed by flow cytometry. The percentage of Annexin V-positive/7-AAD-negative fraction is indicated in the density plot. (d) The percentage of Annexin V-positive/7-AAD-negative fraction summarized in a bar graph. The data are means ± s.d. (**P<0.01,t-test;n=3). (e,f) AML-12 cells were infected with lentiviruses expressing the indicated shRNAs and treated with TGF-β1 for 18 h under serum-starved conditions. Cell lysates were immunoblotted with antibodies against apoptotic markers such as anti-cleaved caspase-3 or anti-PARP. Expression of β-actin was used as a loading control. All data are representative of at least three independent experiments. Figure 7: SMAD6 or A20 knockdown enhances TGF-β1-induced apoptosis. ( a – d ) AML-12 cells were infected with lentiviruses expressing the indicated shRNAs and treated with TGF-β1 for 36 h under serum-starved conditions. ( a ) Cells were stained with propidium iodide (PI) and analysed by flow cytometry The percentages of the subG1 fraction are indicated. ( b ) The percentages of the subG1 fraction are summarized in a bar graph. The data are means ± s.d. (** P <0.01, *** P <0.001 compared with ‘shGFP with TGF-β1(+)’, t -test; n =3). ( c ) Cells were immediately stained with Annexin V and 7-AAD, and analysed by flow cytometry. The percentage of Annexin V-positive/7-AAD-negative fraction is indicated in the density plot. ( d ) The percentage of Annexin V-positive/7-AAD-negative fraction summarized in a bar graph. The data are means ± s.d. (** P <0.01, t -test; n =3). ( e , f ) AML-12 cells were infected with lentiviruses expressing the indicated shRNAs and treated with TGF-β1 for 18 h under serum-starved conditions. Cell lysates were immunoblotted with antibodies against apoptotic markers such as anti-cleaved caspase-3 or anti-PARP. Expression of β-actin was used as a loading control. All data are representative of at least three independent experiments. Full size image To further demonstrate that the increased TGF-β1-mediated apoptosis in A20 knockdown AML-12 cells is due to sustained activation of the TRAF6-TAK1-p38/JNK pathway, we treated the indicated cells with specific inhibitors of TAK1 (5Z-7-oxozeaenol), JNK (SP600125), or p38 MAPK (SB203580) ( Fig. 8 ). After obtaining optimal concentrations of the inhibitors in AML-12 cells ( Fig. 8a ), we examined cell deaths in A20 knockdown AML-12 cells in the presence of TGF-β1 after pre-treatment of each inhibitor for 30 min. Treatment of TAK1 or p38 MAPK inhibitors profoundly inhibited TGF-β1-induced apoptosis of A20 knockdown AML-12 cells ( Fig. 8b,c ). That is, treatment of TAK1 or p38 MAPK inhibitors significantly reduced the increased subG1 fraction of A20 knockdown AML-12 cells. The JNK inhibitor, SP600125, did not cause this effect ( Fig. 8b,c ). These results indicate that sustained activation of the TRAF6-TAK1-p38 MAPK pathway is responsible for TGF-β1-induced apoptosis which is increased in A20 knockdown AML-12 liver cells. Also, these findings suggest that the TGF-β1-induced noncanonical activation of TRAF6-TAK1-JNK is involved in other cellular functions, but not apoptosis. 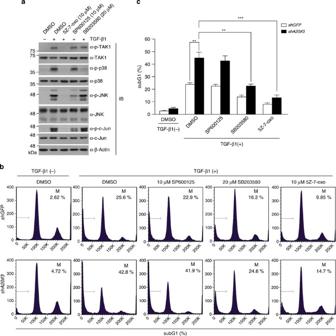Figure 8: TAK1 and p38 MAPK are involved in cell deaths ofA20knockdown cells. (a) AML-12 cells were pre-treated with 10 uM 5Z-7-oxozeaenol (5Z-7-oxo; TAK1 inhibitor), 10 uM SP600125 (JNK inhibitor), or 20 uM SB203580 (p38 MAPK inhibitor) for 30 min and subsequently treated with TGF-β1 for 30 min. The activity of each inhibitor was monitored through detecting expression of phospho-TAK1, phospho-JNK (or phospho-c-Jun), or phospho-p38 MAPK by immunoblotting (IB), respectively. The optimal concentrations of each inhibitor were obtained by repeating these experiments several times. DMSO-containing buffers were used as a negative control. (b) AML-12 cells expressing GFP-specific shRNA or A20-specific shRNA (shA20#3) were pre-treated with each inhibitor for 30 min and subsequently treated with TGF-β1 for 36 h under serum-starved conditions. Cells were analysed by flow cytometry and the percentage of subG1 fraction indicated. (c) Percentages of the subG1 fraction are summarized in a bar graph. The data are means ± s.d. (**P<0.01, ***P<0.001,t-test;n=3). Figure 8: TAK1 and p38 MAPK are involved in cell deaths of A20 knockdown cells. ( a ) AML-12 cells were pre-treated with 10 uM 5Z-7-oxozeaenol (5Z-7-oxo; TAK1 inhibitor), 10 uM SP600125 (JNK inhibitor), or 20 uM SB203580 (p38 MAPK inhibitor) for 30 min and subsequently treated with TGF-β1 for 30 min. The activity of each inhibitor was monitored through detecting expression of phospho-TAK1, phospho-JNK (or phospho-c-Jun), or phospho-p38 MAPK by immunoblotting (IB), respectively. The optimal concentrations of each inhibitor were obtained by repeating these experiments several times. DMSO-containing buffers were used as a negative control. ( b ) AML-12 cells expressing GFP-specific shRNA or A20-specific shRNA (shA20#3) were pre-treated with each inhibitor for 30 min and subsequently treated with TGF-β1 for 36 h under serum-starved conditions. Cells were analysed by flow cytometry and the percentage of subG1 fraction indicated. ( c ) Percentages of the subG1 fraction are summarized in a bar graph. The data are means ± s.d. (** P <0.01, *** P <0.001, t -test; n =3). Full size image Hepatic depletion of SMAD6 causes liver damage To verify the inhibitory role of Smad6 in the TGF-β1-TRAF6-TAK1-p38/JNK pathway in an animal model system, we generated mice with acute liver-specific depletion of SMAD6 by injecting adenoviruses expressing SMAD6 shRNA (Ad-SMAD6i). Adenonviruses expressing nonspecific RNAi (Ad-US) were used as a negative control. Highly increased phosphorylation levels of TAK1, p38 MAPK and JNK were observed in hepatic SMAD6 knockdown mice ( Fig. 9a ). 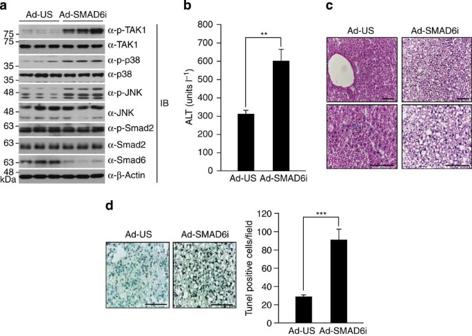Figure 9:SMAD6knockdown mice show liver damage. Mice were injected with adenoviruses expressing shRNAs targetingSMAD6(Ad-SMAD6i), which caused substantial and specific knockdown ofSMAD6in liver. Adenoviruses expressing non-specific RNAi (Ad-US) were used as a control. (a) Mice infected with Ad-US or Ad-SMAD6i were sacrificed and the livers were lysed by homogenization, and immunoblotted with the indicated antibodies. (b) Serum alanine aminotransferase (ALT) levels in mice infected with Ad-US and Ad-SMAD6i. The data are means ± s.e.m. (**P<0.01,t-test;n=5). (c) H&E staining of livers isolated from the mice infected with Ad-US and Ad-SMAD6i. Scale bar, 100 μm. (Magnification; x200-upper, × 400-lower). (d) Livers of the mice infected with Ad-US and Ad-SMAD6i were used for a TUNEL assay. Scale bar, 100 μm. Maginification; × 400. TUNEL-positive cells were quantified and described in a bar graph. The data are means ± s.e.m.(***P<0.001,t-test;n=5). All data are representative of at least three independent experiments. Figure 9: SMAD6 knockdown mice show liver damage. Mice were injected with adenoviruses expressing shRNAs targeting SMAD6 (Ad-SMAD6i), which caused substantial and specific knockdown of SMAD6 in liver. Adenoviruses expressing non-specific RNAi (Ad-US) were used as a control. ( a ) Mice infected with Ad-US or Ad-SMAD6i were sacrificed and the livers were lysed by homogenization, and immunoblotted with the indicated antibodies. ( b ) Serum alanine aminotransferase (ALT) levels in mice infected with Ad-US and Ad-SMAD6i. The data are means ± s.e.m. (** P <0.01, t -test; n =5). ( c ) H&E staining of livers isolated from the mice infected with Ad-US and Ad-SMAD6i. Scale bar, 100 μm. (Magnification; x200-upper, × 400-lower). ( d ) Livers of the mice infected with Ad-US and Ad-SMAD6i were used for a TUNEL assay. Scale bar, 100 μm. Maginification; × 400. TUNEL-positive cells were quantified and described in a bar graph. The data are means ± s.e.m. (*** P <0.001, t -test; n =5). All data are representative of at least three independent experiments. Full size image We next examined whether acute reduction of the hepatic SMAD6 gene affects liver function. Mice with reduced hepatic Smad6 expression displayed greater increase in liver damage, compared with the control group, as measured by serum alanine transaminase (ALT) levels ( Fig. 9b ) and detected by H&E staining ( Fig. 9c ). Liver injury is often accompanied by the apoptosis of hepatocytes. The number of TUNEL-positive apoptotic cells was greatly increased in the hepatic SMAD6 knockdown group ( Fig. 9d ). These results indicate that Smad6 is a critical regulator of liver homoeostasis, and a possible regulatory mechanism is the negative regulation of TGF-β1-induced TRAF6-TAK1-p38/JNK activation. Here we define a novel function of Smad6 as a negative regulator of the noncanonical TGF-β1-TRAF6-TAK1-p38 MAPK/JNK signalling pathway. We show that Smad6, immediately induced in response to TGF-β1 in AML-12 and primary hepatocytes, inhibits TGF-β1-induced TRAF6 polyubiquitination through recruiting the A20 deubiquitinating enzyme, thereby suppressing subsequent TAK1-p38 MAPK/JNK activation. Also, Smad6 inhibited TGF-β1-induced AP-1-mediated reporter activity which reflects JNK activation whereas it did not inhibit Smad-specific CAGA-reporter activity. Our findings shed new light on the function of Smad6 in TGF-β1 signalling, showing that Smad6, but not Smad7, participates in the negative regulation of noncanonical TGF-β signalling. Our results also support a previous report that Smad7 is a positive regulator of the noncanonical TGF-β1-TRAF6-TAK1-p38 MAPK/JNK pathway [30] . Smad7 may act as a scaffold protein in the TGF-β1-TRAF6-TAK1 pathway by binding TAK1 and p38 MAPK [30] , [47] . This is consistent with our results that SMAD7 knockdown decreased the phosphorylation levels of TAK1, p38 MAPK, and JNK. This is the first report that Smad6 recruits the A20 deubiquitinating enzyme, but not CYLD, to negatively regulate the noncanonical TGF-β1-TRAF6-TAK1-p38 MAPK/JNK pathway. Both the A20 and CYLD proteins were originally identified as negative regulators of TNF-α/IL-1β-induced NF-κB signalling that deubiquitinated various targets such as RIP1, TRAF6, TRAF2 and NEMO [31] , [35] , [48] , [49] . In this study, we reveal that A20 recruitment to TβRI-TRAF6 in the presence of TGF-β1 essentially requires Smad6, and subsequently deubiquitinates K63-linked TRAF6 polyubiquitination, resulting in the decrease of TAK1 and p38 MAPK/JNK phosphorylation and AP-1-mediated reporter activity. In certain aspects, this role of Smad6 is likely to be similar to those of ABINs and TAX1BP1, known as A20 adaptors in the inhibition of NF-κB activity in the TNF-α signalling pathway [50] , [51] . ABINs and TAX1BP1 bind to target substrates such as NEMO and RIP1 through their ubiquitin binding domain (UBD) in the TNF-α pathway and recruit the ubiquitin editing enzyme A20, resulting in the deubiquitination of their K63-linked polyubiquitination [50] , [51] . In particular, ABIN proteins as well as A20 are induced by TNF-α, eventually forming a negative feedback loop of the TNF-α pathway [50] . Therefore, these A20 adaptors, binding to ubiquitinylated targets, determine the specificity of diverse cellular substrates for A20. Acting as an adaptor for A20, Smad6 may determine the specificity in inhibiting the noncanonical TGF-β1-TRAF6-TAK1-JNK/p38 MAPK pathway through recruiting A20 to K63-linked polyubiquitinated TRAF6. The differences between ABINs, TAX1BP1 and Smad6 is that Smad6 is induced by TGF-β1 and does not have a UBD domain. Furthermore, our findings suggest that A20 acts as an important regulatory protein in the canonical TGF-β signalling pathway as well as noncanonical TRAF6-TAK1-p38 MAPK/JNK pathway, because A20 knockdown cells showed decreased Smad2 phosphorylation. Therefore, it should be worth investigating the detailed functions of A20 in the canonical TGF-β pathway. A recent report indicated that CYLD decreases stability of Smad3 in a glycogen-synthase kinase3-β (GSK3β)-Hsc70-interacting protein (CHIP)-dependent manner via deubiquitinating Akt in lung fibrotic tissue and mouse lung cells, suggesting that CYLD is a negative regulator of the TGF-β-Smad pathway [52] . However, we did not observe this in CYLD -specific knockdown AML-12 cells, likely due to the differences in cellular context. The physiological importance of the Smad6-A20 axis in the noncanonical TGF-β1-TRAF6-TAK1-p38 MAPK/JNK pathway was supported by lentiviral shRNA-mediated cell-based analysis and animal models with SMAD6 or A20 knockdown by an acute liver-specific adenoviral shRNA system. In particular, immunoblot analysis and treatment of TAK1 and p38 MAPK inhibitors showed that TGF-β1-mediated apoptosis through the noncanonical TGF-β signalling pathway requires TRAF6-TAK1-p38 MAPK ( Fig. 8 ). In contrast, treatment of a JNK inhibitor did not reduce the apoptotic cell deaths of SMAD6 or A20 knockdown AML-12 cells, implying that the TGF-β1-TRAF6-TAK1-JNK pathway is involved in other cellular function, but not apoptosis. In addition, hepatic depletions of SMAD6 and A20 in an animal model increased TAK1 and p38 MAPK phosphorylation as well as apoptotic cell death of liver tissue ( Fig. 9 and Supplementary Fig. S9 ). Interestingly, these results regarding A20 knockdown hepatic depletion, added a new anti-apoptotic mechanism of A20 inhibiting TGF-β1-mediated apoptosis of hepatocytes, compared to those previously showing a protective role of A20 in the liver [53] , [54] , [55] . A20 has been reported to carry out multiple hepatoprotective functions through anti-inflammatory, anti-apoptotic and pro-proliferative effects in hepatocytes [53] , [54] , [55] . The anti-apoptotic function of A20 has been reported to be due to disruption of caspase-8 activation [56] . Our finding suggests that A20 acts as an anti-apoptotic protein through blocking noncanonical TGF-β1-mediated apoptosis in liver cells. Particularly noteworthy is the fact that decreased phosphorylation of Smad2, which was detected in A20 knockdown AML-12 mouse liver cells, was not observed in the liver extracts of A20 knockdown mice. This may be due to differences between liver extracts and the AML-12 mouse cell line, since liver extracts contain many different cell types including Kupffer cells, hepatic stellate cells, and hepatocytes. However, we still do not understand the exact mechanism of how liver apoptosis is detected in an A20-depleted animal model without TGF-β1 treatment. We speculate that Kupffer cells, the resident marcophages of the liver, may play an important role in liver apoptosis in the A20 knockdown animal model. Infection of liver-specific adenoviruses may cause inflammatory responses and initial apoptosis in the infected sites to subsequently recruit innate inflammatory cells including Kupffer cells. As previously reported about hepatocyte cell death [57] , infiltrated Kupffer cells may promote the activation of hepatic stellate cells which further develop into myofibroblasts. The activated myofibroblasts may secrete TGF-β1, which eventually amplify liver apoptosis in the A20 knockdown animal model. Our present findings also prompted us to investigate whether other E3 ubiquitin ligases are involved in the inhibition of TGF-β1-induced TRAF6 polyubiquitination. We first examined the involvement of the Smurf1 E3 ubiquitin ligase which is involved in the selective degradation of MyD88 through binding to Smad6 (ref. 26 ). However, the ubiquitination pattern of TRAF6 was not affected in SMURF1 knockdown cells upon TGF-β1 treatment ( Supplementary Fig. S10 ), providing support that the Smad6-A20 axis is specific for deubiquitination of TGF-β1-induced TRAF6 ubiquitination. In addition, our results also imply that A20 might be involved in TGF-β1-mediated anti-inflammatory function. Our group had previously reported that Smad6, which is induced by TGF-β1, negatively regulates the pro-inflammatory TLR4 signalling pathway through direct binding to Pellino-1 and selective degradation of MyD88 (refs 25 , 26 ). TRAF6 and RIP1 ubiquitination are involved in the TLR4 signalling pathway and subsequent activation of the NF-κB transcription factor [58] . Therefore, it is possible that A20 may participate in inhibition of the TLR4 pro-inflammatory signal through deubiquitinating TRAF6, and that this deubiquitination requires the adaptor function of Smad6. In addition to the TGF-β1-TRAF6-TAK1-p38 MAPK/JNK pathway, several noncanonical TGF-β signalling pathways exist, including the phosphoinositide 3-kinase (PI3K)-Akt-mTOR pathway, the small GTPase Rho, Rac and Cdc42, and the Ras-ERK pathway [5] , [6] , [7] , [8] , [9] , [10] , [11] , [12] , [13] . However, it is unknown how these other noncanonical TGF-β signalling pathways are negatively regulated. It is possible that Smad6 is also involved in the negative regulation of these pathways by recruiting different enzymes depending on the cellular context or which noncanonical TGF-β pathway is activated. Of course, we do not exclude the possibility that Smad7 or other proteins are responsible for the negative regulation of other noncanonical TGF-β signalling pathways. In conclusion, our results reveal the molecular mechanism of negative regulation of the TGF-β1-mediated activation of the TRAF6-TAK1-p38 MAPK/JNK pathway. We demonstrate that TGF-β1-induced Smad6 is a key protein that controls TRAF6 polyubiquitination through recruitment of the A20 deubiquitinating enzyme. Therefore, modulation of this Smad6-A20 axis may be a promising target in the regulation of apoptosis, cell migration, anti-inflammation, and epithelial-mesenchymal transition (EMT) related to the noncanonical TGF-β-induced activation of the TAK1, p38 MAPK and JNK pathway. Plasmids Full-length mouse Flag-TRAF6 complementary DNA (cDNA) and Flag-tagged full length human A20 cDNAs were kind gifts from Dr Jaewhan Song (Yonsei University, Korea). Plasmids encoding different regions of the TRAF6 protein (Flag-TRAF6-D1, Flag-TRAF6-D1/D2, Flag-TRAF6-D3, Myc-TRAF6-CC, Myc-TRAF6-TRAF) were amplified from full-length Flag-TRAF6 cDNA by PCR and subcloned into the EcoRI and NotI sites of the pcDNA3-Flag vector (Invitrogen) or into the EcoRI and SalI sites of the pCS3MTBX-6xMyc vector. Flag-Smad6-MH1-like, Flag-Smad6-linker, Flag-Smad6-MH2, and Flag-Smad6-FL [26] were re-subcloned into the EcoRI and XhoI sites of the pcDNA3-HA vector (Invitrogen). Plasmids encoding domains of the A20 protein (Flag-A20-OTU, Flag-A20-ZFs) were amplified from full-length Flag-A20 cDNA by PCR and subcloned into the EcoRI and XhoI sites of the pcDNA3-Flag vector (Invitrogen). Wild type His-ubiquitin (His-Ub), His-UbK48, and His-UbK63 were previously described [25] . Full-length human Smad7 cDNA was cloned into the EcoRI and XhoI sites of the pcDNA-HA vector. A catalytic inactive A20 point mutant (A20(C103A)), ZF4 mutant (Y614A/F615A), ZF7 mutant (F770A/G771A), and the shRNA-resistant mutant Smad6 were generated using the QuikChange Mutagenesis kit (Stratagene). PCR-generated portions of all constructs were verified by sequencing. PCR primer sequences are described in Supplementary Table S1 . The (CAGA) 12 -Luc luciferase reporter plasmid [59] was kindly provided by Dr Suntaek Hong (Gacheon University, Korea). Cell culture and reagents CMT-93 murine intestinal epithelial cells, human embryonic kidney 293 (HEK293) cells were maintained in DMEM with 10% FBS (GIBCO-BRL). AML-12 alpha mouse liver cells were maintained in DMEM/Ham’s F-12 nutrient mixture (GIBCO) with 10% FBS, 100 nM Dexamethasone (Sigma), ITS premix (BD). Prior to TGF-β1 treatment, AML-12 or CMT93 cells were starved overnight in medium containing 0.5% FBS. The following antibodies were used for immunoblot analysis; mouse anti-HA (16B12, Covance, dilution ratio 1:1,000), rabbit anti-Smad7 (3894-1, Epitomics, 1:500), mouse anti-A20 (59A426, eBioscience, 1:1,000), anti-HA-HRP (Roche, 1:1,000), anti-Ub FK2-HRP (BML-PW0150, Enzo Life Science, 1:1,000), anti-K-63-specific Ub-HRP (BML-PW0605, Enzo Life Science, 1:1,000). Mouse anti-c-Myc (sc-40, 1:1,000), rabbit anti-TRAF6 (sc-7221, 1:1,000), rabbit anti-TAK1 (sc-7162, 1:1,000), rabbit anti-Smurf1 (sc-25510, 1:1,000), mouse anti-CYLD (sc-74435, 1:1,000), rabbit anti-TβRI (sc-402, 1:1,000) were purchased from Santa Cruz Biotechnology. Rabbit anti-p-TAK1 (#4531, 1:500), rabbit anti-TAK1 (#4505, 1:1,000), rabbit anti-p-p38 (#9211, 1:1,000), rabbit anti-p38 (#9212, 1:1,000), rabbit anti-p-JNK (#9251, 1:1,000), rabbit anti-JNK (#9252, 1:1,000), rabbit anti-p-Smad2 (#3101, 1:1,000), rabbit anti-Smad2 (#5339, 1:1,000), rabbit anti-Smad6 (#9519, 1:1,000), rabbit anti-A20 (#5630, 1:1,000), rabbit anti-PARP-1 (#9542, 1:1,000), rabbit anti-cleaved-Caspase3 (#9661, 1:1,000) were purchased from Cell Signalling. Mouse anti-Flag (F3165, 1:1,000), rabbit anti-Flag (F7425, 1:2,000) and mouse anti-β-actin (A5316, 1:5,000) were obtained from Sigma. Mouse anti-His (ab18184, 1: 1,000) was obtained from Abcam. Recombinant human TGF-β1 was obtained from HumanZyme, Inc. Annexin V-FITC (556547) and Propidium Iodide (PI, 51-66211E) were purchased from BD Bioscience, and 7-AAD was obtained from eBioscience. The TAK1 inhibitor (5Z-7-oxozeaenol, 3064) was purchased from Tocris Bioscience. JNK inhibitor (SP600125, E1-305-0010) was obtained from Enzo Life Science and p38 MAPK inhibitor (SB203580, V1161) was purchased from Promega. Construction of small hairpin RNAs and lentiviral infection The short hairpin RNA (shRNA) sequences specific for endogenous SMAD6 , SMAD7 , A20 or CYLD are described in Supplementary Table S2 . Specific shRNAs were purchased from Mission-shRNA (Sigma). The shRNA sequences specific for SMURF1 were previously described [26] . Lentiviruses expressing each siRNA were produced by a lentiviral packaging system from Invitrogen. A lentivirus expressing a green fluorescence protein (GFP) targeting siRNA sequence was used as a negative control for lentivirus infection. Target cells were infected for 24 h with polybrene (8 μg ml −1 ). After incubation for 24 h, media was changed to complete media. After 1 day, cells were trypsinized and were subjected to puromycin selection. Culture of primary hepatocytes Primary hepatocytes were isolated from 8- to 10-week-old C57BL/6 mice by a collagenase perfusion method as described [46] with minor modifications. Cells were plated with medium 199 (Sigma) supplemented by 10% FBS, 10 units per ml penicillin, 10 mg ml −1 streptomycin, and 10 nM dexamethasone. After attachment, cells were infected with lentiviruses coding various shRNAs overnight. Subsequently, medium was changed to fresh culture medium and then incubated for 48 h. 72 h post-infection, cells were treated with TGF-β1 in serum-starved medium for the indicated times. In vivo ubiquitination assay The ubiquitination assay was described previously [26] . Briefly, cells were treated with TGF-β1 for the indicated times, and harvested in 1 ml PBS containing 5 mM N-ethyl maleimide (NEM). Non-covalent protein interactions. were dissociated with 1% SDS and boiling for 10 min. Samples were diluted ten times with lysis buffer (PBS containing 0.5% Triton X-100, 20 mM HEPES (pH 7.4), 150 mM NaCl, 12.5 mM β-glycerol phosphate, 1.5 mM MgCl2, 10 mM NaF, 2 mM DTT, 1 mM NaOV, 2 mM EGTA, 1 mM PMSF, and protease inhibitor cocktail) and subsequently suspended using a 1 ml syringe. The samples were cleared by centrifugation at 16,000 g for 10 min. For immunoprecipitation, lysates were incubated with protein A/G agarose beads and with anti-TRAF6 (sc-7221, Santa Cruz) or anti-TAK1 (sc-7162, Santa Cruz Biotechnology) antibody at 4 °C for 12–16 h. The beads were washed three times with lysis buffer and immunoprecipitates were separated from the beads by adding 2X sample buffer and boiled and fractioned by SDS–PAGE. SDS–PAGE-separated immunoprecipitates were transferred onto PVDF membranes. The membranes were denatured with denaturation buffer containing 6 M guanidine chloride, 20 mM Tris (pH 7.5), 100 mM PMSF, and 5 mM β-mercaptoethanol at 4 °C for 30 min and washed three times with TBST. The membranes were blocked with 5% BSA and incubated with anti-ubiquitin-HRP antibody (FK2, Biomol). Pull-down and ubiquitination assay by Ni-NTA columns Cells were collected in PBS buffer containing 5 mM NEM. Cells were resuspended in binding buffer (6 M guanidine HCl, 0.1 M Na 2 HPO 4 , 0.1 M NaH 2 PO 4 , 0.01 M Tris (pH 8.0), 10 mM β-mercaptoethanol, 5 mM NEM, 5 mM imidazole) and incubated with Ni-NTA agarose (Qiagen) at 4 °C for 12 h. Ni-NTA-mediated pull-down assays were performed as described [26] . Immunoblotting was performed using anti-Flag, anti-HA antibodies. Expression of the β-actin protein was used as a loading control. Animal experiments and recombinant adenovirus Eight-week-old male C57BL/6 mice were purchased from ORIENT BIO (Korea). Mice were housed in a specific pathogen-free animal facility at the Sungkyunkwan University School of Medicine (12:12 h light-dark cycle). For animal experiments involving adenoviruses, mice were tail vein-injected with recombinant adenovirus (0.1–0.5 × 10 9 pfu per mice). 4 days post injection, animals were fasted for 16 h with free access to water. Plasma alanine transaminase (ALT) was measured by DRI-CHEM 4000i (FUJI FILM). All procedures were approved by the Sungkyunkwan University School of Medicine Institutional Animal Care and Use Committee (IACUC). Adenoviruses expressing a nonspecific RNAi control (US), SMAD6i, A20i were generated as described [60] . The RNAi sequences specific for endogenous SMAD6 and A20 are described in Supplementary Table S2 . TUNEL assay Mice were infected with Ad-US, Ad-SMAD6i, or Ad-A20i. Four days post injection, animals were fasted for 16 h and anaesthetized for liver isolation. Livers were stained with hematoxylin and eosin (H&E) for morphological analysis. The TUNEL assay was performed in frozen tissue sections using a standard histological protocol. The sections were permeabilized with Triton X-100 at 4 °C for 2 min and flooded with terminal deoxynucleotidyl transferase and digoxigenin-dUTP reaction buffer (TUNEL) reagent for 60 min at 37 °C. The percentage of apoptotic cell deaths was quantified by counting TUNEL-positive cells among 500 hepatocytes under a light microscope. Transfection and reporter assay Plasmids were transiently transfected into HEK293 using PEI (Polyethyleneimine). Lipofectamine 2000 (Invitrogen) was used for CMT-93 and AML-12 cells. siRNAs were reverse-transfected using Lipofectamine RNAiMAX. Cells were treated for the indicated time with TGF-β1 (5 ng ml −1 ). Luciferase activity was performed with a dual-luciferase reporter assay system (Promega). All experiments were independently repeated at least three times with similar results. Immunofluorescence assay and subcellular fraction Cells were fixed in cold methanol for 7 min, followed by blocking (5% BSA) and incubation with primary antibodies at room temperature for 3 h. Anti-TRAF6 (sc-8409, Santa Cruz, 1:50) antibody and anti-A20 (#5630, Cell Signalling 1:100), anti-TβRI (sc-402, Santa Cruz, 1:50) were used to detect co-localization. After five washes in PBS, coverslips were incubated at room temperature for 3 h with the following secondary antibodies: Alexa fluor-488-conjugated goat anti-rabbit IgG (Invitrogen, 1:100, for anti-A20 or anti-TβRI antibodies), Alexa fluor-594-conjugated donkey anti-mouse IgG (Invitrogen, 1:100, for anti-TRAF6 antibody). Coverslips were stained with DAPI (Santa Cruz) and mounted on a glass slide. Cells were examined with a laser-scanning confocal microscope (Nikon A1Rsi). All images were captured with a CFI Plan Apochromat VC objective lens (60 × /1.40 Oil) at a resolution of 512 × 512 using digital zooming. All images were stored as ND or JPG2000 files, which are standard formats for a Nikon A1Rsi confocal microscope. For subcellular fractionation, the ProteoExtract Subcellular Proteome Extraction Kit (Calbiochem, cat. 539790) was used. Apoptosis analysis For Annexin V/7-AAD staining, cells were collected using trypsin, washed with Annexin V binding buffer, and incubated with Annexin V-FITC and 7-AAD for 15 min (BD Biosciences). For propidium iodide (PI) staining, cells were fixed in 70% ethanol and incubated with 40 μg ml −1 RNase A for 30 min, followed by incubation in 100 μg ml −1 PI for 30 min. Cell cycle was analysed by fluorescence-activated cell sorting (FACS) analysis using FACScan apparatus (BD Biosciences). All data were analysed using CellQuest Pro software (Becton-Dickinson). Immunoblot and immunoprecipitation For immunoblot analysis, cells were lysed in lysis buffer (1% Triton X-100, 20 mM Hepes at pH 7.4, 150 mM NaCl, 12.5 mM β-glycerol phosphate, 1.5 mM MgCl2, 10 mM NaF, 2 mM DTT, 1 mM NaOV, 2 mM EGTA, 1mM PMSF, protein inhibitor cocktail). Protein extracts were separated by SDS-PAGE, transferred to a PVDF membrane filter, and subjected to immunoblot analysis. For immunoprecipitation, lysates were incubated with protein G agarose beads (Genedepot) at 4 °C for 12 h. Immunocomplexes were washed twice with lysis buffer, and separated from the beads by adding 2X sample buffer and boiling. Immunoblot analysis was performed using the indicated antibodies. Full scans of cropped western blots are provided in Supplementary Fig. S11 . RNA extraction and quantitative real-time RT-PCR Total RNA was isolated using the TRIZOL reagent (Invitrogen). The Superscript kit (Invitrogen) was used for reverse transcription. Primer sequences of the BIM and Gapdh genes are described in Supplementary Table S3 . For quantitative RT-PCR, an iCycler real-time PCR machine and iQ SYBR Green Supermix (Bio-Rad) were used to measure the expression of genes under the following conditions; 45 cycles of 95 °C for 30 s, 62 °C for 30 s, and 72 °C for 30 s. Real-time RT-PCR experiments were performed essentially as described [26] . All reactions were independently repeated at least three times to ensure reproducibility. How to cite this article: Jung, S. M. et al . Smad6 inhibits non-canonical TGF-β1 signalling by recruiting the deubiquitinase A20 to TRAF6. Nat. Commun. 4:2562 doi: 10.1038/ncomms3562 (2013).